Identification of Thymosin β4 as an effector of Hand1-mediated vascular development The bHLH transcription factor Hand1 (Heart and neural crest-derived transcript-1) has a fundamental role in cardiovascular development; however, the molecular mechanisms have not been elucidated. In this paper we identify Thymosin β4 ( Tβ4/Tmsb4x ), which encodes an actin monomer-binding protein implicated in cell migration and angiogenesis, as a direct target of Hand1. We demonstrate that Hand1 binds an upstream regulatory region proximal to the promoter of Tβ4 at consensus Thing1 and E-Box sites and identify both activation and repression of Tβ4 by Hand1, through direct binding within either non-canonical or canonical E-boxes, providing new insight into gene regulation by bHLH transcription factors. Hand1-mediated activation of Tβ4 is essential for yolk sac vasculogenesis and embryonic survival, and administration of synthetic TB4 partially rescues yolk sac capillary plexus formation in Hand1-null embryos. Thus, we identify an in vivo downstream target of Hand1 and reveal impaired yolk sac vasculogenesis as a primary cause of early embryonic lethality following loss of this critical bHLH factor. Hand1 (Heart and neural crest-derived transcript-1) is a class B bHLH factor, critical for the development of three embryologically distinct lineages: trophoblast of the placenta, extraembryonic mesoderm derivatives and cardiomyocytes of the left ventricle and outflow tract myocardium. Hand1 -null embryos arrest in development at around embryonic day 8.0 (E8.0) because of extraembryonic defects [1] , [2] , [3] . Trophoblast giant cells, responsible for establishing the implantation chamber by invasion into the maternal decidua, fail to differentiate from trophoblast precursors of the ecto-placental cone [1] , and the visceral yolk sac lacks defined vasculature and shows extensive haemorrhaging [1] , [3] . Tetraploid aggregation experiments rescued extraembryonic defects, enabling development to E10.5, when chimeric embryos died presenting with cardiac anomalies such as abnormal looping and impaired specification of the ventricular myocardium [1] . However, given the potential contribution from both placental and/or yolk sac defects, the primary cause of lethality of Hand1 mutant embryos has not been determined and, moreover, despite previous identification of differential expression of vascular genes downstream of Hand1 [4] , there is no insight into how Hand1 might function in these lineages at the level of direct downstream targets. To gain mechanistic insight into Hand1 function during development, we screened for potential target genes of Hand1 using representational difference analysis between pools of mRNA from in vitro -differentiated wild-type and Hand1 -null embryoid bodies (EBs) [5] . A number of genes implicated in cell motility and guidance were identified as being differentially expressed in the absence of Hand1 . One such gene, the actin monomer-binding protein, thymosin β4 ( Tβ4/Tmsb4x ), was downregulated in the Hand1 -null background, and both temporally and spatially coexpressed with Hand1 in vivo , notably in the left ventricle and outflow tract of the developing heart at mid-gestation and appropriately mis-expressed in Hand1 -null embryos. TB4, the predominant mammalian isoform of the β-thymosin family, sequesters monomeric actin (G-actin), which is then de-sequestered by profilin to induce rapid filament (F-actin) polymerization. This process underlies the formation of filamentous structures such as lamellipodia to mediate cell movement. Specifically, TB4 has been shown to promote the migration of endothelial and other vasculogenic precursor cells and as such is an important regulator of the closely related processes of vasculogenesis and angiogenesis [6] , [7] , [8] , [9] , [10] . Here, we validate Tβ4 as a legitimate downstream target of Hand1 and investigate the functional role of the Hand1–Tβ4 pathway during embryogenesis. Reporter gene co-transfection experiments, electrophoretic mobility shift assays (EMSAs) and chromatin immunoprecipitation (ChIP) confirm that Hand1 directly binds to upstream sequences proximal to the Tβ4 promoter to confer complex transcriptional regulation, seemingly activating and repressing transcription at different consensus binding sites. We reveal how ectopic administration of TB4 rescues vascular differentiation in Hand1 -null embryonic stem cells and defective yolk sac vasculogenesis in Hand1 -null embryos to prolong survival. Thus, we are able to define an early essential role for Hand1 in regulating yolk sac vessel development with Tβ4 as a downstream mediator of Hand1 vascular function. Tβ4 is bound by Hand1 at conserved E-box and Thing1 sites To validate Tβ4 as a legitimate downstream Hand1 target, we performed a range of transcriptional reporter and DNA-binding assays. The functional Tβ4 promoter has previously been identified as residing between residues −278 and +410, relative to the ATG [11] . We identified two upstream putative Hand1-binding sites, a canonical E-Box site, CACATG (consensus CANNTG; nucleotide positions −1913 to −1908) for the binding of bHLH/E-factor heterodimers and a degenerate E-Box, TCTCTG (nucleotide positions −1691 to −1686), which matches the preferred binding site of HAND1/E-factor heterodimers (consensus NCTCTG [12] ; Fig. 1a ). These binding sites are conserved throughout mammals, such as human, rhesus and dog, but not throughout chicken or lower vertebrates species such as frog and zebrafish, consistent with the evolution of the chorioallantoic and yolk sac placenta ( Fig. 1b ; http://ecrbrowser.dcode.org/ ). An 870-bp fragment (−2002 to −1132) containing E-boxes was placed upstream of a luciferase reporter and minimal promoter and we established point mutation constructs in which single residues within half-sites, previously identified as critical for Hand1 or E-Factor binding (Thing1 mutants 1 and 2; E-Box mutant 1) or as an alternate core residue for E-Factor binding to determine specificity (E-box mutant 2) [12] , were individually mutated ( Fig. 1c ). Accordingly, NIH-3T3 cells, co-transfected with the Tβ4 luciferase construct and full-length Hand1 cDNA, were assayed for luciferase activity. Hand1 was shown to induce a 10-fold activation of Tβ4 expression ( Fig. 1d , P <0.001). Activation was completely abolished by point mutation of the Thing1 box, selectively at the half-site of Hand1 binding ( P <0.01; Fig. 1d ), suggesting that Tβ4 is a direct target of Hand1, with activation occurring, primarily, at the Thing 1 box. In contrast, point mutations in the E-box resulted in increased transcriptional activity (2.6-fold increase for the E-box mutant 1, relative to wild type), indicative of an additional level of transcriptional control, whereby Hand1/E-factor binding at this site can repress transcription ( Fig. 1d ). Mutation of the Hand1-binding half-site within the canonical E-box to an alternate core E-box residue resulted in the greatest increase in transcriptional activity ( Fig. 1d ), indicating a high degree of specificity for Hand1 binding of the specific E-Box within the Tβ4 upstream region. To examine the ability of Hand1 to bind to the Tβ4 regulatory sequence, EMSAs were performed using 26-bp double-stranded oligonucleotides corresponding to the E-box and Thing1 sites, along with 10 flanking nucleotides on either side. In vitro -translated Hand1, as a test for homodimer binding, was shown to shift the migration of both binding site oligos ( Fig. 1e ). The greater intensity of the shifted E-box oligo implies stronger binding at the E-box compared with the Thing1 box ( Fig. 1e ). We then investigated binding of in vitro -translated Hand1 in combination with in vitro -translated E-factor (E12) at the E-box and revealed a resulting band shift comparable to that for an optimal Thing1 box (CGTCTG) [12] positive control ( Fig. 1f ). This was supported by additional EMSAs with in vitro -translated tethered Hand1-E-Factor to further investigate heterodimer binding, which again showed stronger binding at the E-box (ITF2; Fig. 1g ). Significantly, binding was virtually undetectable when oligonucleotides containing half-site point mutations were used ( Fig. 1e ) and excess cold (unlabelled) of either half-site mutant was unable to compete away binding relative to that competed by cold wild-type oligonucleotide ( Fig. 1f,g ). 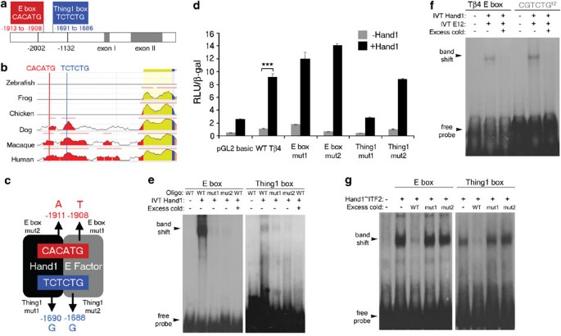Figure 1: Hand1 is a transcriptional regulator of Tβ4. A consensus E-box (CACATG, in red) and Thing1 box (TCTCTG, in blue) are found within a regulatory region upstream of theTβ4promoter (a). Sequence alignment reveals that the Hand1-binding sites proximal to theTβ4promoter are conserved in mammals. Evolutionarily conserved regions are indicated by coloured peaks and represent at least 100 bp of sequence and 70% identity; red peaks represent upstream intergenic regions; yellow peaks represent untranslated regions; blue peak is the first exon of Tβ4 and the salmon region is the intronic sequence (http://ecrbrowser.dcode.org/; (b)). Schematic to illustrate point mutations introduced into the respective half-sites of E-box and Thing1 box; numbers refer to the nucleotide location of each point mutation relative to the ATG of Tβ4 (c). An 870-bp fragment containing the regulatory sequences was placed upstream of a luciferase reporter to assay for transcriptional activity. Luciferase reporter assays indicate a 10-fold activation of a Tβ4 reporter construct by Hand1 (***P<0.001, Student'st-test) (d). Electrophoretic mobility shift assays demonstrate binding of Hand1 to both the E-box and Thing1 boxes within the Tβ4 proximal regulatory sequence, which is abolished by point mutation of E-box residues and severely diminished by point mutation of the Thing1 box (e). EMSA binding of Hand1 and E12 to the E-box within the Tβ4 proximal regulatory sequence compared with an optimal Thing1 Box12(f). Binding of E-box and Thing1 boxes by a tethered Hand1-E-factor (Hand1–ITF2) heterodimer is not competed away by mutant oligonucleotides (as depicted in (c)) containing a point mutation in the half sequence for either E-factor or Hand1 binding (g); IVT controls of empty vector alone are shown in the left-hand lanes for each ofe–g. Error bars indare s.e.m. ofn= mean of three separate transfection experiments, with triplicate wells for each treatment per experiment. IVT,in vitro-translated; RLU, relative light units. Figure 1: Hand1 is a transcriptional regulator of Tβ4. A consensus E-box (CACATG, in red) and Thing1 box (TCTCTG, in blue) are found within a regulatory region upstream of the Tβ4 promoter ( a ). Sequence alignment reveals that the Hand1-binding sites proximal to the Tβ4 promoter are conserved in mammals. Evolutionarily conserved regions are indicated by coloured peaks and represent at least 100 bp of sequence and 70% identity; red peaks represent upstream intergenic regions; yellow peaks represent untranslated regions; blue peak is the first exon of Tβ4 and the salmon region is the intronic sequence ( http://ecrbrowser.dcode.org/ ; ( b )). Schematic to illustrate point mutations introduced into the respective half-sites of E-box and Thing1 box; numbers refer to the nucleotide location of each point mutation relative to the ATG of Tβ4 ( c ). An 870-bp fragment containing the regulatory sequences was placed upstream of a luciferase reporter to assay for transcriptional activity. Luciferase reporter assays indicate a 10-fold activation of a Tβ4 reporter construct by Hand1 (*** P <0.001, Student's t -test) ( d ). Electrophoretic mobility shift assays demonstrate binding of Hand1 to both the E-box and Thing1 boxes within the Tβ4 proximal regulatory sequence, which is abolished by point mutation of E-box residues and severely diminished by point mutation of the Thing1 box ( e ). EMSA binding of Hand1 and E12 to the E-box within the Tβ4 proximal regulatory sequence compared with an optimal Thing1 Box 12 ( f ). Binding of E-box and Thing1 boxes by a tethered Hand1-E-factor (Hand1–ITF2) heterodimer is not competed away by mutant oligonucleotides (as depicted in ( c )) containing a point mutation in the half sequence for either E-factor or Hand1 binding ( g ); IVT controls of empty vector alone are shown in the left-hand lanes for each of e – g . Error bars in d are s.e.m. of n = mean of three separate transfection experiments, with triplicate wells for each treatment per experiment. IVT, in vitro -translated; RLU, relative light units. Full size image Collectively, in vitro DNA-binding analyses not only confer direct binding at specific sites within the Tβ4 proximal 5′ region to Hand1, but for the first time provide evidence for binding within either the preferred Thing1 box or the canonical E-Box, which in turn results in Hand1-mediated differential effects (activation through the Thing1 box and repression through the E-box) on Tβ4 transcription. Tβ4 is a direct in vivo target of Hand1 Definitive in vivo binding of Hand1 to the Tβ4 promoter was demonstrated by ChIP from both EBs and whole embryos. Chromatin from 14-day differentiated wild-type EBs was immunoprecipitated using a polyclonal α-Hand1 antibody and the binding of Hand1 to the Tβ4 regulatory sequence was ascertained by PCR using several primer sets across this region ( Fig. 2a,b ). Chromatin from Hand1 -null EBs was used in parallel as a control for antibody specificity and all PCR products were validated by sequencing. These experiments not only confirm that Hand1 can be induced to bind and regulate Tβ4 transcription in vitro but also show that binding occurred in vivo with EB differentiation. We next sought to extend these studies to verify that the same direct interaction occurred in the developing embryo. Interestingly, the Tβ4 proximal upstream regions were immunoprecipitated using the Hand1 antibody from whole E8.5 embryos but either failed to be immunoprecipitated, in the case of the region containing the Thing1 box, or only relatively weakly (15-fold less by means of scanning densitometry), in the case of the region containing the E-box from E11.5 embryos ( Fig. 2b ), providing additional insight into the temporal control of Hand1-mediated regulation of Tβ4 expression. Western analysis on E8.5 wild-type and Hand1 -null embryos confirmed the specificity of the Hand1 antibody used in ChIP experiments ( Fig. 2c ), which was independently further verified by our inability to ChIP from Hand1 -null EBs. 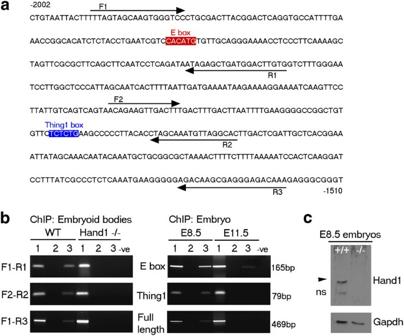Figure 2: Hand1 binds to a region proximal to the Tβ4 promoterin vivo. Regions of the Tβ4 sequence containing either the E-box (F1–R1; forward (F) and reverse (R) primer sequences are underlined with arrowhead for orientation) or the Thing1 box (F2–R2 primer sequences as indicated) were PCR-amplified using indicated primers (a). Chromatin containing the E-box and the Thing1 box was individually immunoprecipitated from wild-type (WT) embryoid bodies but not fromHand1-null embryoid bodies as confirmation of antibody specificity (b). Hand1 binds to the Tβ4 promoter in the E8.5 embryo but only weakly at the E-box of the promoter at E11.5. A 469-bp product containing both binding sites (F1–F3 primer sequences as indicated) could be amplified from both EBs and E8.5 embryos under PCR conditions of reduced stringency. Lanes 1, 2 and 3 refer to input, no antibody control and Hand1 antibody, respectively. Specificity of the antibody used for ChIP was confirmed by western blot analysis of E8.5 WT (+/+) andHand1-null (−/−) embryos (c); black arrowhead highlights specific Hand1 band; ns, nonspecific. Figure 2: Hand1 binds to a region proximal to the Tβ4 promoter in vivo . Regions of the Tβ4 sequence containing either the E-box (F1–R1; forward (F) and reverse (R) primer sequences are underlined with arrowhead for orientation) or the Thing1 box (F2–R2 primer sequences as indicated) were PCR-amplified using indicated primers ( a ). Chromatin containing the E-box and the Thing1 box was individually immunoprecipitated from wild-type (WT) embryoid bodies but not from Hand1 -null embryoid bodies as confirmation of antibody specificity ( b ). Hand1 binds to the Tβ4 promoter in the E8.5 embryo but only weakly at the E-box of the promoter at E11.5. A 469-bp product containing both binding sites (F1–F3 primer sequences as indicated) could be amplified from both EBs and E8.5 embryos under PCR conditions of reduced stringency. Lanes 1, 2 and 3 refer to input, no antibody control and Hand1 antibody, respectively. Specificity of the antibody used for ChIP was confirmed by western blot analysis of E8.5 WT (+/+) and Hand1 -null (−/−) embryos ( c ); black arrowhead highlights specific Hand1 band; ns, nonspecific. Full size image The Hand1–Tβ4 pathway regulates vasculogenesis in EBs Transcriptional and DNA-binding assays identified Tβ4 as a direct target of the transcription factor, Hand1. We sought to establish the functional significance of the Hand1–Tβ4 pathway in vivo , by determining the role of Tβ4 in Hand1-dependent developmental processes. Given the requirement for Tβ4 in coronary vasculogenesis and angiogenesis, we investigated whether reduced levels of TB4 contribute to vascular defects in Hand1 -null embryos. Initially, we made use of Hand1 -null EBs as a surrogate model for vasculogenesis [13] , [14] . Hand1 -null EBs were morphologically indistinct from wild-type EBs and able to undergo differentiation into complex cell types, such as beating cardiomyocytes, and primitive morphogenesis, including vesicle formation and cavitation. We first investigated the relative expression of Hand1 and Tβ4 over a time course of EB differentiation. As wild-type EBs were differentiated in floating culture, expression of Hand1 , first apparent at day 4, became upregulated and reached a peak of expression at day 8. Tβ4 expression was first detected after 6 days of differentiation. Significant upregulation of Tβ4 , followed immediately after Hand1 expression, reached peak level (10 days of differentiation). The lag between the onset of Hand1 expression and upregulation of Tβ4 likely reflects the earlier expression of Hand1 in EB cell lineages that do not express Tβ4 (for example, definitive mesoderm). Appropriate succession of Tβ4 relative to Hand1 in EB differentiation is consistent with the notion that Tβ4 is a bona fide Hand1 target ( Fig. 3a ). Real-time quantitative reverse transcription (qRT)–PCR, over the equivalent time course of both wild-type R1 and Hand1 -null (6.13) EB differentiation, confirmed appropriate downregulation of Tβ4 expression in Hand1 -null EBs ( Fig. 3b–d ), although Tβ4 levels were not completely ablated, suggesting that, during differentiation of the embryo proper, Hand1 is not the only factor regulating Tβ4 gene expression. We then examined expression levels of key vascular genes in Hand1 -null EBs and observed reduced expression of both endothelial (TIE-2; to 4.1%; Fig. 3e ) and smooth muscle (α-smooth muscle actin; α-SMA; to 62.7%) cell markers ( Fig. 3f ). To determine the extent to which the loss of Tβ4, downstream of Hand1, accounted for the reduced expression of these specific vascular markers, EBs were cultured in the presence of 100-ng ml −1 synthetic TB4 from day 4 of differentiation until collection at day 14. Addition of TB4 to the culture medium was sufficient to restore endothelial differentiation, represented by TIE-2 levels, the more severely downregulated marker in the Hand1 -null situation ( Fig. 3e ). α-SMA levels, which were modestly diminished in the absence of Hand1 , were significantly elevated (2.2- to 4.5-fold) beyond control levels, not only in Hand1 -null EBs but also in Hand1 -heterozygous and wild-type EBs ( Fig. 3f ), implying that TB4 is a potent regulator of embryonic smooth muscle cell differentiation. However, as smooth muscle protein levels were not greatly reduced in the Hand1 -null background, it is possible that, in this context, TB4 functions in smooth muscle differentiation in a parallel pathway independent of Hand1. 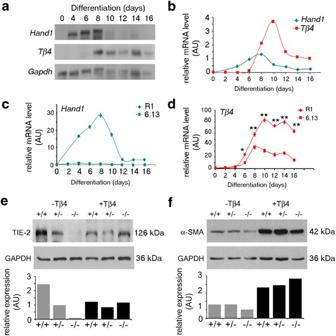Figure 3: Hand1 regulates vascular differentiation in embryoid bodies. Tβ4and Hand1 levels were visualized by northern blotting (a) and quantified relative toGapdhlevels (b). Real-time qRT–PCR was used to measureHand1(c) orTβ4expression (d) during a time course of differentiation in wild-type (R1) andHand1-null (6.13) EBs. Tβ4 levels are significantly downregulated in aHand1-null background (day 6, *P≤ 0.05; days 8–16, **P≤ 0.01; Student'st-test) (d). Western blot analysis showed that vascular markers, both endothelial (e) and smooth muscle (f), are diminished inHand1-null embryoid bodies (EBs), as quantified by scanning densitometry, normalized against GAPDH. Expression levels of these markers, TIE-2 (e) and α-SMA (f), are restored by supplementing the culture medium with synthetic TB4 (+Tβ4). Error bars incanddrepresent s.e.m., wheren= mean of three samples per time point. AU, arbitrary units. Figure 3: Hand1 regulates vascular differentiation in embryoid bodies. Tβ4 and Hand1 levels were visualized by northern blotting ( a ) and quantified relative to Gapdh levels ( b ). Real-time qRT–PCR was used to measure Hand1 ( c ) or Tβ4 expression ( d ) during a time course of differentiation in wild-type (R1) and Hand1 -null (6.13) EBs. Tβ4 levels are significantly downregulated in a Hand1 -null background (day 6, * P ≤ 0.05; days 8–16, ** P ≤ 0.01; Student's t -test) ( d ). Western blot analysis showed that vascular markers, both endothelial ( e ) and smooth muscle ( f ), are diminished in Hand1 -null embryoid bodies (EBs), as quantified by scanning densitometry, normalized against GAPDH. Expression levels of these markers, TIE-2 ( e ) and α-SMA ( f ), are restored by supplementing the culture medium with synthetic TB4 (+Tβ4). Error bars in c and d represent s.e.m., where n = mean of three samples per time point. AU, arbitrary units. Full size image The Hand1–Tβ4 pathway regulates yolk sac vasculogenesis We next investigated the implications of these findings by addressing the role of the Hand1–Tβ4 pathway in the development of the yolk sac vasculature proper. As Hand1 was shown to be expressed in the mesodermal layer of the visceral yolk sac [3] , [4] , as a contributory factor to the haemorrhagic yolk sac phenotype reported in Hand1 -null embryos, we first examined the developing yolk sac vasculature as a potential lineage for Hand1 – Tβ4 coexpression. In situ hybridization revealed Tβ4 expression in the blood islands of the yolk sac at E8.5 ( Supplementary Fig. S1a ) and in developing vessels at E9.5 and E10.5 ( Supplementary Fig. S1b–d ). Whole-mount immunofluorescence, on wild-type embryos, revealed Tβ4 coexpression with Hand1 throughout the yolk sac mesoderm at E8.5 ( Fig. 4a,b ) and in endothelial cells at E8.5 (not shown) and E9.5 ( Fig. 4c ). Tβ4 was not expressed in smooth muscle cells, as revealed at E9.5 ( Supplementary Fig. S2a–d ). Hand1 follows an equivalent pattern of expression at E9.5, exclusively localized within the platelet/endothelial cell adhesion molecule (PECAM)+ endothelium ( Fig. 4d,e ) and absent from the smooth muscle layer of the developing yolk sac vasculature ( Fig. 4f,g ). Interestingly, Hand1 subcellular localization changes from exclusively nuclear at E8.5 to perinuclear at E9.5 (as confirmed by immunostaining with three independent α-Hand1 polyclonal antibodies), with increasing endothelial cell differentiation ( Fig. 4a,b,d and e ), and is downregulated on vascular maturation ( Supplementary Fig. S2e–h ). 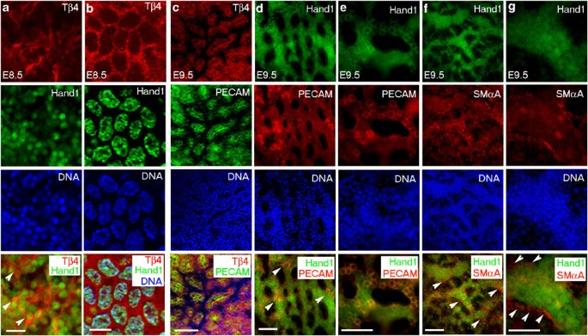Figure 4: TB4 and Hand1 are coexpressed in the developing yolk sac. TB4 is coexpressed with Hand1 in the yolk sac mesoderm at E8.5 as determined by immunostaining with epifluoresence (a) and confocal microscopy (b). White arrowheads ina(merged, bottom panel) highlight Tβ4 and Hand1 double-positive cells. TB4 is expressed in endothelial cells of yolk sac capillaries at E9.5 (c), as detected by coexpression with PECAM (c; panel 4). Hand1 is expressed in yolk sac PECAM+ endothelial cells and becomes localized to perinuclear regions with differentiation of the endothelium (d,e); white arrowheads highlight clusters of Hand1+/PECAM+ endothelial cells ind(merged bottom panel) with a higher magnification view of costained cells within the plexus ine. Hand1 is not expressed in smooth muscle cells at E9.5, as indicated by mutually exclusive localization of Hand1+ cells and those stained for α-smooth muscle actin (αSMA;f,g); white arrowheads highlight αSMA+ cells lining the Hand1+ vascular endothelium at low (f) and high magnification (g). Each top panel label (a–g) refers to the subsequent set of four vertical panels. Scale bars indicate 20 μm (a); 10 μm (b); and 50 μm (c–g). Figure 4: TB4 and Hand1 are coexpressed in the developing yolk sac. TB4 is coexpressed with Hand1 in the yolk sac mesoderm at E8.5 as determined by immunostaining with epifluoresence ( a ) and confocal microscopy ( b ). White arrowheads in a (merged, bottom panel) highlight Tβ4 and Hand1 double-positive cells. TB4 is expressed in endothelial cells of yolk sac capillaries at E9.5 ( c ), as detected by coexpression with PECAM ( c ; panel 4). Hand1 is expressed in yolk sac PECAM+ endothelial cells and becomes localized to perinuclear regions with differentiation of the endothelium ( d , e ); white arrowheads highlight clusters of Hand1+/PECAM+ endothelial cells in d (merged bottom panel) with a higher magnification view of costained cells within the plexus in e . Hand1 is not expressed in smooth muscle cells at E9.5, as indicated by mutually exclusive localization of Hand1+ cells and those stained for α-smooth muscle actin (αSMA; f , g ); white arrowheads highlight αSMA+ cells lining the Hand1+ vascular endothelium at low ( f ) and high magnification ( g ). Each top panel label ( a–g ) refers to the subsequent set of four vertical panels. Scale bars indicate 20 μm ( a ); 10 μm ( b ); and 50 μm ( c – g ). Full size image Rescue of Hand1 vascular defects by synthetic TB4 Importantly, TB4 was significantly downregulated (9.03-fold, P ≥ 0.01) in Hand1 -null yolk sacs to levels equivalent to background (no primary/secondary antibody-alone controls; not shown), as determined by immunostaining ( Fig. 5a–f ) and ImageJ analysis for quantification ( Fig. 5g ). Subsequent immunohistochemistry on Hand1 -mutant embryos indicated a lack of vascular plexus formation in the yolk sacs of mutant embryos as compared with heterozygous littermates at E8.5 ( Fig. 6a,b ). Such defects in yolk sac vasculogenesis coincided, as previously reported [1] , with an arrest in embryonic development. In contrast, wild-type and heterozygous littermate embryos had appropriately turned and developed within a yolk sac containing a well-organized capillary plexus composed of PECAM+ endothelial cells arranged in the characteristic honeycomb pattern ( Fig. 6a ). Intraperitoneal injection of pregnant female mice with TB4 (6 mg kg −1 ) was performed to determine whether defective vasculogenesis in Hand1 -null yolk sacs could be rescued by TB4. Hand1 -null embryos treated with TB4 were recovered at E8.5 in which yolk sacs displayed an appropriately formed capillary network (PECAM immunohistochemistry, Fig. 6c–f ) and in which the embryo had developed beyond the primitive arrested head fold and body axis stage of the conventional mutants. Appropriate uptake of TB4 in the yolk sac vasculature was confirmed by enzyme-linked immunosorbent assay (ELISA) on treated yolk sac tissue, which revealed a significant fivefold elevation in TB4 levels ( Fig. 6g ). In addition, real-time qRT–PCR revealed that reduced Tβ4 expression in Hand1 mutant yolk sacs was elevated beyond the level observed in control Hand1 heterozygotes after administration of synthetic TB4 ( Fig. 6h ); this not only further confirmed appropriate localization of TB4 treatment to the developing yolk sac in utero , but also suggested an autoregulatory effect of TB4 on its own gene expression. In two independent Hand1 -null lines (conventional targeted Hand1 allele and a tTA knock-in to the Hand1 locus), the mutant phenotype at E8.5 is virtually 100% penetrant [1] , [15] , as confirmed in all vehicle-treated mutants examined in this study, suggesting that TB4-rescued mutants do not simply represent Hand1 mutants presenting with a less-severe phenotype. Therefore, we conclude that TB4 is sufficient to rescue vasculogenic defects in the embryonic yolk sac that arise because of an absence of Hand1 . Conventional Hand1 mutants were rarely observed at E9.5 ( n = 1 from 5 litters/49 embryos, expected number=12.5; 25%) and those that could be isolated displayed gross phenotypical defects compared with heterozygous littermates ( Fig. 6i ), leading to resorption ( Fig. 6j ); however, TB4-rescued Hand1 mutants were recovered, but had evidently arrested in development by this stage ( Fig. 6k ). At E9.5, TB4-rescued Hand1 -null embryos were recovered with 16–18 somite pairs, compared with 17–23 in wild-type/heterozygous littermates (based on n = 6 litters), representing a clear progression in development beyond the 8–12 somite pairs observed at E8.5. The E9.5 'rescued' embryos lacked large, blood-filled, vitelline vessels and the accompanying highly organized meshwork of secondary smaller vessels apparent in wild-type yolk sac at the equivalent stage ( Fig. 6l–r ). This suggests that Tβ4 rescued early yolk sac vasculogenesis at E8.5 but was insufficient to rescue angiogenic remodelling of the primary vascular plexus at E9.5 to ensure continued embryonic growth and survival. 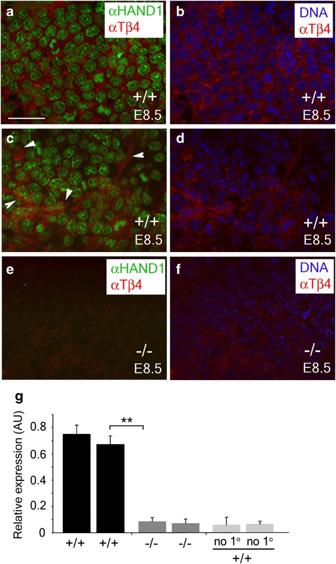Figure 5: TB4 is downregulated inHand1-null yolk sacs. Hand1 and TB4 are coexpressed in the developing vasculature of the yolk sac at E8.5 in wild-type (+/+) embryos (a,c) but not inHand1-null yolk sacs (−/−) (e). TB4 expression is found in the cytoplasm of wild-type embryos as revealed by counterstaining nuclear DNA withbis-benzamide (b,d), but is not detected inHand1-null yolk sacs (f). TB4 is evident in the remodelling vascular plexus (c; highlighted by white arrowheads) in wild-type yolk sacs but significantly downregulated inHand1-null yolk sacs (e–g). Images were captured at equivalent light intensity and filter settings and levels of TB4 were detected inHand1-null yolk sacs as equivalent to background as determined by ImageJ scans of six regions of yolk sac vasculature across two wild-type and twoHand1-null yolk sacs (g). Error bars are s.e.m., wheren= mean ImageJ fluorescence across six regions of yolk sac vasculature per genotype. **P≤ 0.01 (Student's t-test). Scale bar ina, 40 μm (a–f). AU, arbitrary units. Figure 5: TB4 is downregulated in Hand1 -null yolk sacs. Hand1 and TB4 are coexpressed in the developing vasculature of the yolk sac at E8.5 in wild-type (+/+) embryos ( a , c ) but not in Hand1 -null yolk sacs (−/−) ( e ). TB4 expression is found in the cytoplasm of wild-type embryos as revealed by counterstaining nuclear DNA with bis -benzamide ( b , d ), but is not detected in Hand1 -null yolk sacs ( f ). TB4 is evident in the remodelling vascular plexus ( c ; highlighted by white arrowheads) in wild-type yolk sacs but significantly downregulated in Hand1 -null yolk sacs ( e – g ). Images were captured at equivalent light intensity and filter settings and levels of TB4 were detected in Hand1 -null yolk sacs as equivalent to background as determined by ImageJ scans of six regions of yolk sac vasculature across two wild-type and two Hand1 -null yolk sacs ( g ). Error bars are s.e.m., where n = mean ImageJ fluorescence across six regions of yolk sac vasculature per genotype. ** P ≤ 0.01 (Student's t-test). Scale bar in a , 40 μm ( a–f ). AU, arbitrary units. 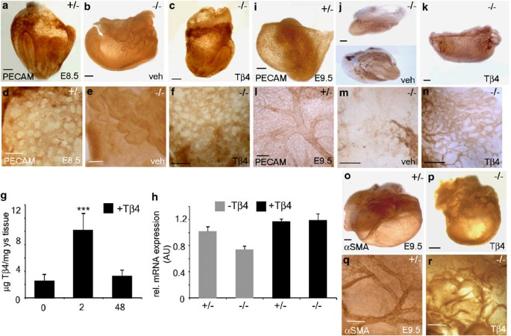Figure 6: TB4 rescues defective yolk sac vasculogenesis inHand1-null mutants. Whole-mount immunohistochemistry was performed on Hand1-null embryos and heterozygote littermate controls at E8.5 (a–f) and E9.5 (i–r) using PECAM (a–f;i–n) and αSMA (o–r) antibodies to visualize the yolk sac capillaries and smooth muscle, respectively. A lack of appropriate capillary plexus formation (vasculogenesis) is evident in Hand1-null embryos (b,e), compared with heterozygous littermates at E8.5 (a,d). Intraperitoneal (i.p.) injection of pregnant females with TB4 rescued the yolk sac vasculogenic defects and an appropriately formed vascular plexus is observed at E8.5 (c,f). ELISA revealed a significant fivefold increase in yolk sac TB4 levels 2 h after injection (6 mg kg−1, i.p.) of pregnant females (g); error bars are s.e.m., wheren= mean protein concentration from six yolk sacs per treatment. ***P<0.001 (Student'st-test). TB4 concentration returns to control (uninjected or 2 h PBS) level by 48 h after injection, consistent with a mean terminal half-life of 1.8–2.1 h (human Phase IA study, RegeneRx). qRT–PCR revealed that diminishedTβ4expression inHand1mutant yolk sacs was elevated to beyond the level observed in controlHand1heterozygotes after administration of synthetic TB4 (h). Angiogenic remodelling (i,l) and smooth muscle recruitment (o,q) occurred in heterozygous embryos by E9.5 but Tβ4–rescued embryos arrested in development before undergoing these processes (k,n,p,r). Hand1-null embryos are seldom recovered at E9.5. An embryo collected at this stage presented with a primitive, avascular yolk sac and was observed to undergo resorption (j,m). TB4 injection had no effect on the yolk sac vasculature of wild-type or heterozygous embryos and hence is not shown. Scale bars indicate 150 μm (a–c); 100 μm (d–f); 250 μm (i–k); 150 μm (l–n); 250 μm (o–r). AU, arbitrary units; ys, yolk sac. Full size image Figure 6: TB4 rescues defective yolk sac vasculogenesis in Hand1 -null mutants. Whole-mount immunohistochemistry was performed on Hand1-null embryos and heterozygote littermate controls at E8.5 ( a – f ) and E9.5 ( i – r ) using PECAM ( a–f ; i–n ) and αSMA ( o–r ) antibodies to visualize the yolk sac capillaries and smooth muscle, respectively. A lack of appropriate capillary plexus formation (vasculogenesis) is evident in Hand1-null embryos ( b , e ), compared with heterozygous littermates at E8.5 ( a , d ). Intraperitoneal (i.p.) injection of pregnant females with TB4 rescued the yolk sac vasculogenic defects and an appropriately formed vascular plexus is observed at E8.5 ( c , f ). ELISA revealed a significant fivefold increase in yolk sac TB4 levels 2 h after injection (6 mg kg −1 , i.p.) of pregnant females ( g ); error bars are s.e.m., where n = mean protein concentration from six yolk sacs per treatment. *** P <0.001 (Student's t -test). TB4 concentration returns to control (uninjected or 2 h PBS) level by 48 h after injection, consistent with a mean terminal half-life of 1.8–2.1 h (human Phase IA study, RegeneRx). qRT–PCR revealed that diminished Tβ4 expression in Hand1 mutant yolk sacs was elevated to beyond the level observed in control Hand1 heterozygotes after administration of synthetic TB4 ( h ). Angiogenic remodelling ( i , l ) and smooth muscle recruitment ( o , q ) occurred in heterozygous embryos by E9.5 but Tβ4–rescued embryos arrested in development before undergoing these processes ( k , n , p , r ). Hand1-null embryos are seldom recovered at E9.5. An embryo collected at this stage presented with a primitive, avascular yolk sac and was observed to undergo resorption ( j , m ). TB4 injection had no effect on the yolk sac vasculature of wild-type or heterozygous embryos and hence is not shown. Scale bars indicate 150 μm ( a–c ); 100 μm ( d–f ); 250 μm ( i–k ); 150 μm ( l–n ); 250 μm ( o–r ). AU, arbitrary units; ys, yolk sac. Full size image Real-time qRT–PCR on E8.5 yolk sacs from Hand1 heterozygous and homozygous mutants confirmed 'rescue' of vascular gene expression during yolk sac vessel development after treatment with synthetic TB4 ( Fig. 7 ). Elevated levels of Vegf , Flt1 and Pecam expression in Hand1 -null yolk sacs, consistent with that observed previously [4] , were returned to control levels after TB4 treatment ( Fig. 7a ). Western analysis on lysates from E8.5 yolk sacs for PECAM expression confirmed the real-time qRT–PCR data. PECAM protein was elevated in the Hand1 -null background, but returned to control levels as observed in heterozygous littermates after TB4 treatment ( Fig. 7b ). The expression data suggest that vascular genes and proteins, such as PECAM, are mis-regulated in a Hand1 -null background, with compensatory increases occurring in yolk sac endothelial cells in the absence of appropriate remodelling and plexus formation. 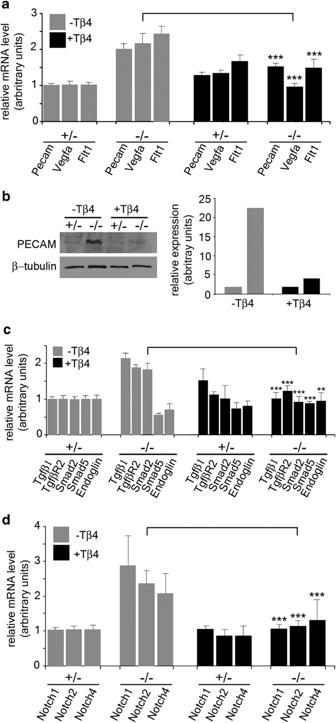Figure 7: TB4 restores appropriate vasculogenic gene and protein expression in theHand1-null yolk sac. Real-time qRT–PCR on E8.5 yolk sacs demonstrated the mis-expression of vascular genes inHand1homozygous mutant yolk sacs (−/−) compared with heterozygous yolk sacs (+/−) and their restoration after treatment with synthetic TB4. Elevated levels ofVegf,Flt1andPecamexpression inHand1-null yolk sacs were returned to control levels after TB4 treatment (a). Differential expression ofPecamwas confirmed at the protein level by western blotting with α-PECAM on lysates from E8.5Hand1-heterozygous andHand1-null yolk sacs treated with either vehicle (−TB4) or TB4 (+TB4): TB4 treatment restored elevated PECAM levels inHand1mutants to control levels as determined in heterozygous littermates (b). Genes implicated in vasculogenic endothelial cell proliferation, migration and differentiation (Tgfβ1, TgfβrII, Smad5,EndoglinandSmad2) were also rescued to the control levels observed inHand1heterozygous yolk sacs (c). Elevated expression ofNotch1,2and4in mutants was also reduced to control levels after administration of TB4, to restore appropriate VEGF signalling and vascular patterning (d). Error bars are s.e.m., wheren= mean of three separate qRT–PCR experiments on three pooled yolk sacs carried out in triplicate. **P<0.01; ***P<0.001 (Student'st-test). Figure 7: TB4 restores appropriate vasculogenic gene and protein expression in the Hand1 -null yolk sac. Real-time qRT–PCR on E8.5 yolk sacs demonstrated the mis-expression of vascular genes in Hand1 homozygous mutant yolk sacs (−/−) compared with heterozygous yolk sacs (+/−) and their restoration after treatment with synthetic TB4. Elevated levels of Vegf , Flt1 and Pecam expression in Hand1 -null yolk sacs were returned to control levels after TB4 treatment ( a ). Differential expression of Pecam was confirmed at the protein level by western blotting with α-PECAM on lysates from E8.5 Hand1 -heterozygous and Hand1 -null yolk sacs treated with either vehicle (−TB4) or TB4 (+TB4): TB4 treatment restored elevated PECAM levels in Hand1 mutants to control levels as determined in heterozygous littermates ( b ). Genes implicated in vasculogenic endothelial cell proliferation, migration and differentiation ( Tgfβ1, TgfβrII, Smad5 , Endoglin and Smad2 ) were also rescued to the control levels observed in Hand1 heterozygous yolk sacs ( c ). Elevated expression of Notch1 , 2 and 4 in mutants was also reduced to control levels after administration of TB4, to restore appropriate VEGF signalling and vascular patterning ( d ). Error bars are s.e.m., where n = mean of three separate qRT–PCR experiments on three pooled yolk sacs carried out in triplicate. ** P <0.01; *** P <0.001 (Student's t -test). Full size image Genes encoding members of upstream TGFβ-signalling pathways, Tgfβ1 and TgfβrII , with associated expression of either Smad5 and Endoglin ( Fig. 7c ), which, at this comparatively early stage, are indicative of endothelial cell proliferation and migration, or Smad2 ( Fig. 7c ), which functions in endothelial cell differentiation during vasculogenesis (reviewed by Gaengel et al . [16] ), were also rescued to the levels observed in control Hand1 heterozygous yolk sacs. In addition, expression of Notch1 , 2 and 4 ( Fig. 7d ) was also reduced to control levels after administration of TB4, suggesting appropriate modulation of VEGF-signalling and vascular patterning (reviewed by Roca and Adams [17] ). Consistent with the TB4-mediated 'rescue' being restricted to vasculogenesis at E8.5, we did not observe changes in expression of genes encoding members of the platelet-derived growth factor (PDGF)-B–PDGFRβ pathway, known to have a key role in mural cell recruitment during angiogenesis. [16] During development, the yolk sac gives rise to blood and the earliest vessels, and functions as the developmental circulatory system to sustain early embryonic life. The initial requirement for complex yolk sac vasculature is then superseded by the placenta, which takes over the supply of maternally derived nutrients and oxygen to the rapidly developing fetus. The bHLH transcription factor Hand1 is fundamentally required for development of both the yolk sac and trophoblast cells of the placenta and, at later stages, in cardiac looping morphogenesis and ventricular specification of the embryo proper. However, to date, as both placentation [1] and extraembryonic mesoderm/yolk sac defects [3] , [4] contribute towards the phenotype of Hand1 -null embryos, it has not been possible to determine the individual contribution of each component or which is primarily responsible for the early embryonic lethality. Moreover, the molecular target genes for Hand1 and downstream effectors, which orchestrate these essential embryonic events, have not been defined. Here, we identify Thymosin β4 as a bona fide target of Hand1 and define a specific physiological role for the Hand1–Tβ4 axis in regulating yolk sac vasculogenesis. Yolk sac vessel anomalies in Hand1 -null embryos manifest at an earlier stage (E8.5) than almost all other reported yolk sac mutants, in which defective angiogenesis and vascular remodelling (PDGF receptors [18] , Neuropilin-1 [19] , Ets-related factor, TEL [20] , LBP-1a [21] , α-5β1 integrin [13] ) or smooth muscle cell recruitment (Erk–5 (ref. [22] )) is evident between E9.0–10.0. We report the first rescue of extraembryonic vascular defects in any context to date, such that administration of synthetic TB4 during pregnancy is sufficient to restore vasculogenesis to Hand1 -null embryonic yolk sacs. The fact that TB4 treatment enabled the recovery of Hand1 -null mutants as late as E9.5 implicates impaired yolk sac vasculogenesis as a contributing factor to the early lethality in Hand1 -null embryos. However, failure of development beyond E9.5 in 'rescued' mutants suggests an absolute requirement for Hand1 in other critical aspects of embryonic development, such that TB4-treated embryos likely die because of a combination of abnormal trophoblast/placenta formation and failed later-stage yolk sac remodelling. A recent study targeting Hand1 specifically in extraembryonic mesoderm [23] resulted in lethality at stages equivalent to those previously reported for systemic Hand1 knockouts [3] , [4] . Loss of Hand1 in extraembryonic mesoderm suggests that the role of Hand1 in the yolk sac anlage is critical for embryonic viability and may represent the primary cause of lethality in Hand1 -null mutants. Yolk sac defects in Hand1 -null mutants have previously been attributed to impaired remodelling of the vascular plexus and defective recruitment of smooth muscle cells to the endothelial network [4] . These events occur after vasculogenesis, and are indicative of the fact that Hand1 mutants in this earlier study survived to a more advanced stage (E9.5), as compared with our null embryos (E8.5), having been generated by distinct targeting to derive an alternate mutant allele and maintained on a different genetic background [4] . Precedent for allele-specific targeting generating phenotypes with a different stage of onset and varying severity exists for a number of genes, including the cardiac transcription factor Gata4 [24] , [25] , whereby the variation is likely due to genetic modifier or off-target effects. Impaired angiogenesis was associated with an upregulation in Vegf , Ang1 and Ephrin B2 at E9.5 but without insight into the functional downstream pathway(s) or any direct effects on gene expression [4] . Consistent with these later-stage findings, we observed an upregulation in components of the Vegf , Tgfβ and Notch pathways in Hand1 -null yolk sacs at E8.5, suggesting that Hand1 may also be required for suppression of specific cohorts of vascular genes at earlier stages. Importantly, whereas mis-expression of these factors may underlie defective angiogenesis and mural cell recruitment at E9.5 [4] , each of these specific pathways is also critical for endothelial cell migration, proliferation and differentiation during vasculogenesis [16] and their mis-expression can account for the earlier Hand1 -null yolk sac phenotype we observe at E8.5. At a biochemical level, we reveal that Tβ4 is a direct target of Hand1 and demonstrate the ability of this transcription factor to both activate and repress transcription of TB4 by binding at alternate E-box sites closely positioned within proximal sequences upstream of the functional promoter [11] . Our ChIP data suggest binding of the Thing1 degenerate E-box in the Tβ4 proximal regulatory region at E8.5 to cause activation of Tβ4 , and, subsequently at E11.5, a relatively stronger binding of Hand1 to the E-box than to the Thing1 box within the same Tβ4 upstream element to mediate repression of Tβ4 . It was previously proposed that the inhibitory activity of HAND1 may be attributed to multiple mechanisms, such as its ability to function as a co-repressor, the presence of a repression domain and its ability to sequester E-factors in an inactive complex [26] . In this study, point mutation of the Tβ4 proximal E-box led to increased transcriptional activity, supporting the possibility that Hand1 represses, at least in the case of Tβ4 , by direct DNA binding rather than limiting the availability of other bHLH factors through sequestration. Interestingly, a point mutation specifically in the predicted Hand1-binding half-site of the Thing1 box, but not the E-factor-binding half, abolished transcriptional activation. This is the first example, of which we are aware, regarding the significance of half-site binding in the context of bHLH heterodimer formation. However, in light of our EMSA data ( Fig. 1e–g ), which revealed an equivalent reduction in DNA binding for point mutants of either the Hand1 or E-Factor half-site within the Thing1 box, further studies are required to determine putative DNA-binding independent mechanisms that might underlie the differential transcriptional regulation by Hand1. These data, collectively, are consistent with previous results that show that HAND1 can function as a negative or positive regulator of transcription [26] , [27] . Evidence of vascular gene repression by Hand1 and the seemingly contradictory lack of vasculogenesis in Hand1 -null embryos, suggest that attempts to compensate for the loss of Hand1 with elevated vascular signalling contributes to the impaired vasculogenesis phenotype in mutants. Therefore, Hand1, through activation and repression of Tβ4 , seems to contribute to the fine-tuning of the vasculogenic response in the yolk sac in a coordinated manner to ensure appropriate temporal and spatial regulation of vessel development. Provascular genes are repressed at times when vessel formation is not desired and transcriptional activation occurs with the onset of vasculogenesis. With specific reference to the ChIP data presented, we speculate that, in the case of TB4, such Hand1-induced temporal regulation at critical stages, between E8.5 and E11.5, may be mediated by a shift in binding from the E-box to the Thing1 box. This remains to be fully proven. We herein implicate TB4 in the process of yolk sac vasculogenesis, downstream of Hand1. TB4 has recently been recognized for its ability to promote coronary vessel development and angiogenesis, both in the embryo and in the adult through neovascularization to promote cardiac repair [28] , [29] . Direct parallels can be drawn between development of the yolk sac, coronary and gut vasculature, which differ from the vasculogenesis that occurs in most other tissues. In all three cases, vascular precursors arise from a mesoderm-derived epithelium, the yolk sac mesothelium [18] , the epicardium [28] , [30] , [31] and the serosal mesothelium [32] . It may be that the provasculogenic role of Tβ4 is restricted to targeting mesothelial tissues specifically for the induction of new vessel formation. Notably, both the epicardium and serosal mesothelium retain vasculogenic potential in the adult [28] , [33] , which, in the case of the epicardium, can be induced by Tβ4 [28] . Given the significant therapeutic potential of Tβ4 in the cardiac setting [6] , [34] and its current use in clinical trials for conditions such as venous stasis and diabetic foot ulcers, epidermolysis bullosa and third-degree skin burns ( http://www.regenerx.com/wt/page/clinical_trials ), all of which require restoration of the subepidermal vascular bed, an understanding of the molecular pathways within which Tβ4 signals is vital, although it is currently lacking. Upstream regulation of Tβ4 has not previously been demonstrated and the identification of Hand1 in this context is significant. It remains a possibility that Hand1 additionally regulates Tβ4 expression at later embryonic stages, perhaps at time points when Tβ4 is required for coronary vasculogenesis. Similarly, very little is known regarding the developmental genes and key signalling pathways that are downstream of Hand1/Tβ4. We reveal mis-expression of a number of provascular genes and their rescue by Tβ4, implicating Tβ4 in pathways that directly or indirectly regulate endothelial cell proliferation, migration and differentiation. However, it remains to be determined whether Hand1–Tβ4 functions to regulate additional factors in vascular development and how these molecular cues may be used during neovascularization and adult cardiac repair. Plasmids The Tβ4 luciferase reporter construct consisting of an 870-bp product, corresponding to a regulatory region upstream of the Tβ4 promoter (−2002 to −1132, relative to ATG), was PCR-amplified from mouse cDNA with the introduction of Kpn I (5′) and Bgl II (3′) sites. The cut product was ligated into Kpn I/ Bgl II-digested pGL2-Basic. For deletion constructs, the promoter fragment was digested with Xmn I/ Bgl II (Δ E-box, 770 bp) or Dra I/ Bgl II (Δ Thing1 box, 460 bp) and ligated into Sma I/ Bgl II-digested pGL2-Basic. Point mutation constructs were created from the full-length reporter construct by site-directed mutagenesis, using QuickChange XL (Stratagene) and appropriate oligonucleotides to introduce the E-box or Thing1-box mutations illustrated in Figure 1 . pcDNA3Hand1 was constructed by ligating an Nde I(filled in)/ Xho I fragment of full-length Hand1 into pcDNA3 and the tethered heterodimer Hand1–ITF2 was constructed by ligating a Bgl I/ Hin dIII fragment of Hand1 and Pst I/ Xba I fragment of ITF2 separated by a peptide tether [GT(G 3 -S 7 ) 4 GGGT] 2 [35] into pCMVFlag. Bioinformatics An ensemble ( http://www.ensembl.org/index.html ) reference sequence, Tmsb4x [NM_021278], chrX: 163643026-163646250, containing the murine upstream regulatory region of Tβ4 (–2002 to −1132, relative to ATG), was entered into the Evolutionary Conserved Regions (ECR) browser at http://ecrbrowser.dcode.org/ . The mouse sequence was used as a base against alignments with sequenced genomes from six species. The graphical output was a smooth conservation plot based on ECRs of 100 nucleotides and 70% identity. Mouse strain The Hand1 -null mouse strain used in this study was generated by homologous recombination in embryonic stem cells using a gene targeting construct derived from a 129sv genomic library with a 5′ arm (5.7 kb Bam HI/ Kpn I fragment) and 3′ arm (2.6 kb Xho I/ Not I fragment) flanking a neomyocin resistance cassette to replace from 0.3 kb upstream of exon I of the Hand1 gene to 0.4 kb downstream of the translation stop codon in exon 2. The targeting generated a functionally null allele in male chimera mice, which was transmitted through the germ line [1] . Experiments on animals were carried out under UK Home Office Project Licenses PPL 70/6086 and PPL 70/6946 in accordance with the UK Animals (Scientific Procedures) Act 1986. Tβ4 rescue in Hand1 -null embryos Timed matings were established between Hand1 -null heterozygous mice. Eighteen pregnant females were injected intraperitoneally with 6 mg kg −1 TB4 (RegeneRx) in 0.1 ml PBS and 12 with vehicle at E4.5 and E6.5 (E8.5 and E9.5 for collection only). Embryos were collected at E8.5 or E9.5 and prepared for immunohistochemistry or qRT–PCR analysis. Western blotting Western blotting was performed using standard methods with antibodies against TIE-2 and PECAM (both from Santa Cruz, diluted 1:200), SMαA (1:1000) and Hand1 (1:500, both from Sigma), and β-tubulin and GAPDH (both from Chemicon, diluted 1:1000). Scanning densitometry was performed and signal quantified using ImageJ. EMSAs EMSAs were carried out essentially as described previously [12] . Briefly, in vitro -translated Hand1, E12 and tethered Hand1–ITF2 heterodimer were incubated with 32 P-labelled oligonucleotide in binding buffer at room temperature for 30 min. Unlabelled oligonucleotide (50-fold excess) was used in the competition binding assays. Binding reactions were run on a 6% tris-borate-edta polyacrylamide gel, which was dried and subjected to autoradiography. Culture of floating EBs Embryonic stem cell lines (wild-type +/+; heterozygous +/−; homozygous −/−) were maintained in culture, as previously described. [36] Cells at approximately 80% confluence were trypsinized and collected in leukaemia inhibitory factor-free differentiation medium. Cells (~10 6 ) were transferred to 100 mm non-coated bacteriological plates and maintained in floating culture for 16 days, with daily feeding. For TB4 rescue experiments, TB4 was added to the culture medium at 100 ng ml −1 after the fourth day of differentiation until collection. EBs were collected at various time points, washed twice in PBS and snap-frozen. Poly(A) RNA was isolated using the Micro-Fast Track 2.0 kit (Invitrogen) and protein extraction was performed using RIPA buffer and a standard protocol. Reporter transactivation assays NIH-3T3 cells, cultured under standard conditions, were transfected using Effectene reagent as described previously [37] . Briefly, duplicate wells were transfected with a reporter (the Tβ4 promoter or mutated versions thereof, upstream of luciferase in pGL2 basic), along with either 250 ng pcDNA3-Hand1 or 250 ng pcDNA3 and a pCMV-β-galactosidase (β-gal) vector to normalize for transfection efficiency. Luciferase and β-gal activity were assayed 48 h after transfection as described [37] ; following normalization, differences in RLU/β-gal were analysed using a Student's t -test. Each transfection experiment was performed three times and a representative data set is shown for each. ChIP Wild-type and Hand1-null EBs were collected after 14 days of differentiation, and washed twice in PBS. E8.5 and E11.5 embryos were dissected in PBS containing 0.3% Triton X-100. Tissues were immediately cross-linked for 3 h at room temperature in ChIP fix (1.8% formaldehyde, 50 mM HEPES pH7.9, 1 mM EDTA, 1 mM EGTA, 100 mM NaCl and 0.09% (v/v) butyric acid), homogenized in lysis buffer and sonicated. A volume of 60 μg of chromatin lysate was used per immunoprecipitation with 10 μg of anti-Hand1 antibody (Sigma) in ChIP dilution buffer at 4°C overnight. A no-antibody procedure was performed in parallel as a control. Immune complexes were pulled down with Protein A/G beads, washed, resuspended in TE (10 mM Tris, 5 mM EDTA, pH 8.0), the cross-links reversed overnight at 65°C and the DNA purified. ChIP and no-antibody samples were assayed by PCR using primers designed to amplify regions of the Tβ4 proximal regulatory region, as illustrated in Figure 2 . ELISA for Tβ4 Pregnant wild-type female mice were injected with Tβ4 (6 mg kg −1 in PBS) or vehicle control either 48 or 2 h before collection of E8.5 embryos. Protein extracts were prepared from six yolk sacs of each treatment group using the RIPA method. A volume of 10 μg of total protein was assayed in duplicate using a Tβ4 ELISA kit (Immundiagnostik), according to manufacturer's instructions. Mean Tβ4 concentration was calculated and significance determined using a Student's t -test. Whole-mount immunohistochemistry Embryos were dissected in sterile PBS, within their yolk sacs, and fixed in 4% (w/v) paraformaldehyde for 2 h at room temperature. Embryos were treated with 3% (v/v) hydrogen peroxide in PBS to block endogenous peroxidase activity and permeabilized by incubation for 3×15 min in PBT ×0.3 (PBS containing 0.3% Triton X-100), 2×15 min in PBT ×0.5 (PBS containing 0.5% Triton X-100), followed by two further 15 min incubations in PBT ×0.3 . Embryos were blocked for 1 h at room temperature in PBT ×0.3 /BR (2% blocking reagent (Roche) in PBT ×0.3 ). The blocking solution was replaced with antibody, diluted in PBT ×0.3 /BR for overnight incubation at 4°C (biotinylated rat anti-PECAM, BD Pharmingen, 1:50; rabbit anti-α-SMA, Abcam, 1:150). Following two rinses in PBT ×0.3 and three 1 h washes in PBT ×0.5 , embryos were blocked for 1 h at room temperature in PBT ×0.3 /BR and incubated overnight with biotinylated anti-rabbit antibody (Dako, 1:100), diluted in BR ×0.3 (except for PECAM staining, using a biotinylated primary antibody when the second day washes and incubation with biotinylated secondary antibody were omitted). After two rinses in PBT ×0.3 and three 1 h washes in PBT ×0.5 , embryos were incubated with diluted streptavidin–horseradish peroxidase complex (diluted in PBT ×0.3 /BR), washed three times in PBT ×0.3 , rinsed in PBS and developed using a 3,3′-Diaminobenzidine Liquid Substrate System (Sigma). After imaging, DNA was prepared from embryos for genotyping, with primers as shown in Supplementary Table S1 [1] . RNA in situ hybridization of embryonic yolk sacs Whole-mount in situ hybridization of embryos retained within the yolk sac was performed, as previously described [4] using a Tβ4 3′UTR riboprobe. qRT–PCR of EBs and yolk sac vascular genes For real-time qRT–PCR analysis of Hand1 and Tβ4 through differentiation, wild-type (R1) and Hand1 -null (6.13) EBs were collected at days 2, 4, 6, 8, 10, 12, 14 and 16, snap-frozen and total RNA extracted using an RNeasy kit (Qiagen). For yolk sac vascular genes, embryos were collected at E8.5, yolk sacs were snap-frozen and DNA was extracted from embryos. After genotyping, four yolk sacs per genotype/treatment group were pooled and total RNA was extracted. Linear amplification of mRNA was performed using a Microarray Target Amplification kit (Roche), according to manufacturer's instructions. qRT–PCR analysis was performed on an ABI 7000 Sequence Detector (Applied Biosystems) using SYBR Green (Applied Biosystems). Data were normalized to Hprt1 expression and gene expression was calculated using the ΔΔ C t method [38] . P -values were obtained using Student's t -test ( n = 9). Primers sequences were obtained from Primer Bank ( http://pga.mgh.harvard.edu/primerbank ), and are shown in Supplementary Table S1 . Yolk sac immunofluorescence Whole-mount embryos with yolk sacs intact were dissected and fixed as described above. Embryos were removed before yolk sacs were blocked and incubated with primary antibody as described above (Cy3-conjugated αSMA (Sigma, 1:200), anti-PECAM (BD Pharmingen, 1:50), ×3 anti-Hand1 (Santa Cruz, 1:50; Sigma, 1:200; and an additional polyclonal anti-Hand1, a kind gift from Dr Orford, 1:200) or anti-TB4 (Immundiagnostik, 1:100)). After washing, as above, the following secondary antibodies were used (all diluted 1:200): Alexa 594-conjugated anti-rabbit (Tβ4), Alexa 488-conjugated anti-rabbit (TB4), Alexa 488-conjugated anti-goat (Hand1) or Alexa 488-conjugated anti-rat (PECAM)). Nuclei (DNA) were stained with 5 mg ml −1 of bis-benzamide (Hoechst 33342; Sigma) in PBS for 10 min at room temperature. Quantitative measures of levels of fluorescence were determined on images captured at equivalent light intensities and filter settings by an investigator blinded to genotype using ImageJ software and compared against no-primary/secondary antibody-alone controls. Accession numbers: NM_021278 . How to cite this article: Smart, N. et al . Identification of Thymosin β4 as an effector of Hand1-mediated vascular development. Nat. Commun. 1:46 doi: 10.1038/ncomms1041 (2010).